Vesicles derived via AP-3-dependent recycling contribute to asynchronous release and influence information transfer Action potentials trigger synchronous and asynchronous neurotransmitter release. Temporal properties of both types of release could be altered in an activity-dependent manner. While the effects of activity-dependent changes in synchronous release on postsynaptic signal integration have been studied, the contribution of asynchronous release to information transfer during natural stimulus patterns is unknown. Here we find that during trains of stimulations, asynchronous release contributes to the precision of action potential firing. Our data show that this form of release is selectively diminished in AP-3b2 KO animals, which lack functional neuronal AP-3, an adaptor protein regulating vesicle formation from endosomes generated during bulk endocytosis. We find that in the absence of neuronal AP-3, asynchronous release is attenuated and the activity-dependent increase in the precision of action potential timing is compromised. Lack of asynchronous release decreases the capacity of synaptic information transfer and renders synaptic communication less reliable in response to natural stimulus patterns. Synaptic information processing depends on the amplitude and time course of neurotransmitter release from presynaptic terminals. While the peak amplitude of release is generally thought to determine information transfer, the time course of the release has significant impact on the precision and reliability of signalling [1] , [2] . These two key parameters of neurotransmitter release and synaptic signalling depend on quick and reliable vesicle recycling. Therefore, modifications in vesicle endo and exocytosis can lead to altered synaptic interactions and information coding in neural circuits [3] , [4] . Spontaneous transmitter release is independent of presynaptic action potentials [5] . In contrast, presynaptic firing triggers synchronous and asynchronous release. These various forms of neurotransmitter release have distinct effects on postsynaptic signal processing. While synchronous release provides rapid communication with postsynaptic neurons, asynchronous release modulates postsynaptic excitability within relatively long periods of time. Hence, it can alter action potential firing patterns and could influence neuronal network reverberations [6] , [7] , [8] . Asynchronous release has also been suggested to play a key role in temporal summation and action potential timing [7] , [9] . In the present study we aimed to determine how asynchronous release is influenced by changes in presynaptic stimulus patterns and how this activity-dependent process alters postsynaptic action potential firing. Vesicles can recycle either directly from the plasma membrane via clathrin-dependent endocytosis, or via intermediate endosomes [10] . Vesicle recycling via endosomes is also called ‘bulk endocytosis’ as several vesicles simultaneously recycle into a single endosome. This mode of vesicle recycling is primarily active during intense neuronal activity [11] . But how does this mode of vesicle recycling influence synaptic signalling and information transfer? The adaptor protein 3 (AP-3) regulates the vesicle formation from endosomes in this distinct endocytotic pathway. In the absence of AP-3, the loss of tetanus-sensitive release augmented calcium-independent release and modified the vesicle pool refilling [12] , [13] . We investigated how the neuronal-specific deletion of AP-3 alters synaptic communication and information transfer at hippocampal mossy fibre–CA3 pyramidal cell synapses. This synapse is an ideal model to investigate this question, as it operates with a relatively large vesicle pool [14] , [15] and during place cell activity hippocampal granule cells fire at a high rate [16] . These physiological parameters are ideal for bulk endocytosis, as it is a highly activity-dependent process [11] and is more likely to occur in larger presynaptic terminals [17] . Synaptic vesicles can be sorted into various pools based on their availability for release (reviewed in the study by Alabi and Tsien [18] ) and the type of neurotransmitter release to which they contribute (reviewed in the study by Ramirez and Kavalali; and Kaeser and Regehr [19] , [20] ). It has been reported that clathrin-dependent vesicle recycling preferentially replenishes the readily releasable pool (RRP) and bulk endocytosis refills the reserve pool [21] . Furthermore, recent evidence also indicate vesicle exchange between different pools: a recycling pool made of releasable vesicles can participate in the refilling of the RRP, as well as exchange vesicles with reserve pool [18] , [22] . In contrast, the relative contribution of vesicles generated via different recycling pathways to various forms of neurotransmitter release is largely unexplored. Interestingly, functional heterogeneity among synaptic vesicles has been suggested based on their molecular composition [23] , [24] . Though it is not observed universally, emerging evidence suggest that two distinct modes of neurotransmitter release—synchronous and asynchronous, utilize vesicles differing in their DOC2, TRPV1, synaptobrevin 2 and VAMP4 content [25] , [26] . However, this issue is currently debated as other findings point to the existence of a single pool of vesicles that support both types of release [27] , [28] . Since AP-3 has been suggested to play a key role in the generation of vesicles with specific membrane protein content [29] , [30] , the deletion of AP-3 potentially could lead to the alteration of a specific form of neurotransmitter release. We aimed to determine the physiological role asynchronous release plays in postsynaptic signal integration. The selective elimination of vesicles derived via the bulk endocytotic pathway using knockout (KO) animals lacking neuronal AP-3 [31] diminished asynchronous release without compromising the synchronous component. We found that upon stimulation of the mossy fibre inputs with natural stimulation patterns, the precision of postsynaptic firing of CA3 pyramidal cells is attenuated due to the selective loss of asynchronous release. Information transfer is significantly augmented by asynchronous release underlining the important role of various forms of neurotransmitter release in synaptic information processing. Complex firing pattern influences action potential precision Granule cells and other principal cells in the hippocampus fire at high rates when animals enter the corresponding place field of a neuron [16] . Mossy fibre terminals are often referred to as a ‘detonator synapse’ because bursts can effectively discharge postsynaptic CA3 pyramidal cells [32] . First, we aimed to determine whether high frequency bursts occur randomly or are preferentially embedded in other firing frequencies at hippocampal mossy fibre synapses. We analyzed in vivo granule cell firing patterns to identify regions where granule cells fire with bursts ( in vivo granule firing patterns are a generous gift from Dr György Buzsáki (NYU, New York, NY, USA)). A correlation between the probability of burst firing and the lengths of the preceding silence is not linear, which indicates that the appearance of bursts is not random ( Supplementary Fig. 2A,B ). Two peaks were observed: the first peak corresponds to double bursts, and the second to the mean preceding silence period of 105 ms (~10 Hz). Thus, high frequency bursts preferentially were embedded in a low frequency activity in the theta range. We selected short stimulus trains ( Fig. 1a ) corresponding to this peak to investigate how the history of presynaptic firing alters postsynaptic coding. We quantified two key parameters of postsynaptic coding: probability of action potential generation and temporal precision. 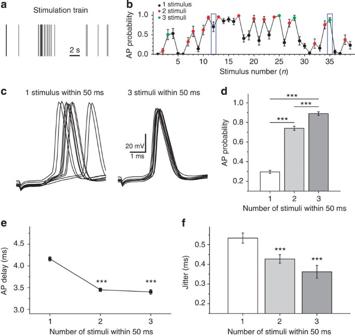Figure 1: Temporal precision of postsynaptic action potentials enhanced after natural short burst stimulation. (a) Example of natural stimulation train and corresponding probability of evoked postsynaptic action potentials. (b) Blue boxes indicate position of individual stimulus (1) and last stimulus in a 50-ms burst of three stimuli (3). Examples of postsynaptic spikes evoked by these stimuli are shown inc(10 traces included). Note the difference in the action potential jitter between single stimulation (one stimulus within 50 ms, left) and stimulation after two preceding stimuli (three stimuli within 50 ms, right). (d) Action potential probability, delay (e) and jitter (f) as a function of the number of stimuli within 50 ms. Note that action potential probability significantly increases with the number of stimuli, while spike delay and jitter become significantly smaller after burst stimulation (two to four stimuli,n=18). Error bars show s.e.m. ***P<0.001, Student’st-test. Figure 1: Temporal precision of postsynaptic action potentials enhanced after natural short burst stimulation. ( a ) Example of natural stimulation train and corresponding probability of evoked postsynaptic action potentials. ( b ) Blue boxes indicate position of individual stimulus (1) and last stimulus in a 50-ms burst of three stimuli (3). Examples of postsynaptic spikes evoked by these stimuli are shown in c (10 traces included). Note the difference in the action potential jitter between single stimulation (one stimulus within 50 ms, left) and stimulation after two preceding stimuli (three stimuli within 50 ms, right). ( d ) Action potential probability, delay ( e ) and jitter ( f ) as a function of the number of stimuli within 50 ms. Note that action potential probability significantly increases with the number of stimuli, while spike delay and jitter become significantly smaller after burst stimulation (two to four stimuli, n =18). Error bars show s.e.m. *** P <0.001, Student’s t -test. Full size image The probability of action potential generation was calculated from responses to every stimuli in the train, based on 10 responses evoked by repetitive presentations of the same stimulation pattern ( Fig. 1b ). The probability of postsynaptic action potential firing varied greatly between 0 and 1. The probability of action potential firing increased significantly with the number of preceding stimuli (0.33±0.02 after single stimulus, 0.72±0.02 after two and 0.87±0.03 after three to four stimuli ( Fig. 1d )). Temporal precision is defined by the delay of postsynaptic action potentials and the variance of this parameter—action potential jitter. These two parameters can influence the efficiency and reliability of neuronal information coding, particularly during high frequency stimulation. Action potential delay was significantly longer if there were no preceding stimuli in the previous 50 ms and spike delay was shortened by the presence of at least one preceding stimulus ( Fig. 1e ). The magnitude of action potential jitter was negatively correlated with the number of stimuli used in a 50 ms time-window. The variability of action potential delay showed an activity-dependent alteration in response to in vivo stimulus patterns, action potential jitter was significantly smaller when more than one stimuli was used within 50 ms (0.38±0.03 ms and 0.28±0.02 ms, respectively, Fig. 1c,f ). These results suggest that the temporal precision of information coding is significantly influenced by the pattern of incoming stimuli. Asynchronous release alters action potential jitter Asynchronous release is known to influence action potential timing and postsynaptic signal integration [7] , [9] . We aimed to determine whether this form of neurotransmitter release could play a role in the activity-dependent changes in action potential timing we observed in response to in vivo stimulus patterns. Asynchronous release occurs in an action potential-dependent manner when neurotransmitter release is delayed and unsynchronized. We investigated the parameters of this release using short 20 Hz trains to stimulate mossy fibre terminals. Recorded responses had two clear components: large, fast rising excitatory postsynaptic synaptic currents (EPSCs) associated with each stimulus; and numerous small events prominent during the EPSCs decay phase. These events were observed up to 700 ms after the last stimulus ( Fig. 2a ). Since asynchronous release occurs several tens and even hundreds of milliseconds after action potentials, it relies mainly on slow calcium dynamics arising either from calcium accumulation during repetitive presynaptic firing or from a longer distance between local calcium entry and the site of vesicle fusion [8] , [33] . We applied the membrane permeable slow calcium chelator ethyleneglycol-bis(β-aminoethyl)-N,N,N′,N′-tetra acetoxymethyl ester (EGTA-AM) (100 μM) to confirm the presence of asynchronous release at the synapse after trains of stimuli. Asynchronous release could be reliably detected after 10 evoked events (20 Hz). Following EGTA-AM application, the frequency of asynchronous EPSCs (aEPSCs) was significantly reduced from 8.16±0.75 to 2.85±1.03 Hz ( Fig. 2a,b ). Moreover, total transferred charge during this period of time was also significantly reduced from 3.6±1.1 to 0.5±0.5 pC ( Fig. 2b ). Similarly to our results obtained with in vivo stimulus patterns, action potential jitter decreased as the number of stimuli increased in the train ( Fig. 2c,e ). Conversely, in the presence of EGTA-AM, the precision of spike timing was not dependent on the number of preceding stimuli, suggesting that asynchronous release potentially could play a role in this phenomenon ( Fig. 2d,e ). EGTA-AM has previously been shown to reduce the synchronous component under certain circumstances [34] , [35] , [36] , this effect is most probably associated with multivesicular neurotransmitter release from mossy fibre boutons. Even though we observed a prominent decrease in the rate of short-term facilitation ( Fig. 2a ) and a reduction of AP probability after EGTA-AM application (control: P =0.98±0.02; EGTA-AM: P =0.77±0.06 in response to 5th stimulus), the latter effect was not significant at the end of the train ( Fig. 2f ). Nevertheless the strongest decrease (approximately three times) in AP jitter happened in response to the last three stimuli (black columns, Fig. 2f ). These data support our conclusion that the presence of synchronous release alone (sufficient to trigger postsynaptic AP) is not enough to reduce jitter during stimulation trains. Moreover, if the increase in synchronous release were responsible for dejittering, the AP jitter would not decrease when facilitation is reduced. Such condition could be achieved using high external calcium concentration (increased initial P ) in the artificial cerebrospinal fluid (ACSF) ( Fig. 2g ). In the presence of 6 mM CaCl 2 , facilitation of EPSC amplitudes during 20 Hz stimulation trains was reduced more than three times ( Fig. 2g ), while the frequency of aEPSCs was significantly higher 14±1 Hz ( n =5) and AP jitter was decreasing during the train to the same degree ( Fig. 2h ) as in 2.5 mM CaCl 2 . Therefore, not the amount of release, but rather the specific increase in the asynchronous component seems to be necessary for AP dejittering. 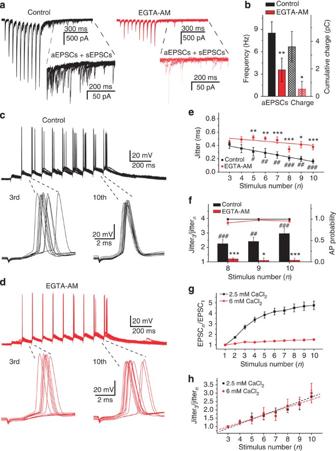Figure 2: Slow calcium chelator EGTA-AM blocks the asynchronous response and prevents spike dejittering. (a) EPSCs evoked by stimulation trains (20 Hz, 10 stimuli) in control conditions (black) and after application of 100 μM EGTA-AM (red), five individual responses are shown. Inserts show expanded 500 ms regions with a mixture of aEPSCs and sEPSCs. (b) Bar graph showing significant reduction in aEPSC frequency and cumulative transferred charge after EGTA-AM application. Examples of postsynaptic spikes evoked by 10 stimuli at 20 Hz in control (black,c) and after EGTA-AM (red,d). Action potentials evoked by the 3rd and 10th stimuli are expanded, 10 responses are shown. Note that action potential jitter calculated within 6 ms after stimulation significantly decreases at the end of the train (c, bottom right) in control conditions, but not after EGTA-AM (d, bottom right). (e) Significant decrease is observed in action potential jitter starting from the fifth stimulus (#P<0.05,##P<0.01 and###P<0.001; Student’st-test), which is abolished in the presence of EGTA-AM (n=7). Significantly larger jitter is present after EGTA-AM application compared with control (*P<0.05, **P<0.01 and ***P<0.001; Student’st-test). (f) AP jitter decreases most profoundly at the end of the stimulation train in control condition (black bars), reaching a threefold decrease by the 10th stimuli. EGTA-AM (red bars) significantly impairs jitter reduction, even though it does not change AP probability (black and red squares) in response to the last three stimuli. Normalized EPSC peak amplitudes (g) and AP jitter (h) recorded at 2.5 mM (black) and 6 mM (red) CaCl2in response to 20-Hz stimulation train. Note that facilitation is more than three times smaller at high calcium concentration (n=25 andn=7 for 2.5 mM and 6 mM CaCl2, respectively), but AP jitter decreases to the same degree (n=8 andn=7 for 2.5 mM and 6 mM CaCl2, respectively). Dashed lines correspond to linear fits of the data. Error bars show s.e.m. Figure 2: Slow calcium chelator EGTA-AM blocks the asynchronous response and prevents spike dejittering. ( a ) EPSCs evoked by stimulation trains (20 Hz, 10 stimuli) in control conditions (black) and after application of 100 μM EGTA-AM (red), five individual responses are shown. Inserts show expanded 500 ms regions with a mixture of aEPSCs and sEPSCs. ( b ) Bar graph showing significant reduction in aEPSC frequency and cumulative transferred charge after EGTA-AM application. Examples of postsynaptic spikes evoked by 10 stimuli at 20 Hz in control (black, c ) and after EGTA-AM (red, d ). Action potentials evoked by the 3rd and 10th stimuli are expanded, 10 responses are shown. Note that action potential jitter calculated within 6 ms after stimulation significantly decreases at the end of the train ( c , bottom right) in control conditions, but not after EGTA-AM ( d , bottom right). ( e ) Significant decrease is observed in action potential jitter starting from the fifth stimulus ( # P <0.05, ## P <0.01 and ### P <0.001; Student’s t -test), which is abolished in the presence of EGTA-AM ( n =7). Significantly larger jitter is present after EGTA-AM application compared with control (* P <0.05, ** P <0.01 and *** P <0.001; Student’s t -test). ( f ) AP jitter decreases most profoundly at the end of the stimulation train in control condition (black bars), reaching a threefold decrease by the 10th stimuli. EGTA-AM (red bars) significantly impairs jitter reduction, even though it does not change AP probability (black and red squares) in response to the last three stimuli. Normalized EPSC peak amplitudes ( g ) and AP jitter ( h ) recorded at 2.5 mM (black) and 6 mM (red) CaCl 2 in response to 20-Hz stimulation train. Note that facilitation is more than three times smaller at high calcium concentration ( n =25 and n =7 for 2.5 mM and 6 mM CaCl 2 , respectively), but AP jitter decreases to the same degree ( n =8 and n =7 for 2.5 mM and 6 mM CaCl 2 , respectively). Dashed lines correspond to linear fits of the data. Error bars show s.e.m. Full size image Next, we aimed to determine whether the observed activity-dependent action potential jitter decrease in response to stimulus trains is solely the result of alteration in presynaptic release dynamics. We used glutamate uncaging to mimic the release of 10 identical synaptic events at 20 Hz ( Fig. 3 ). We uncaged glutamate at the close proximity of thorny excrescences of CA3 pyramidal cells using two-photon point illumination. When EPSPs were evoked at 20 Hz, action potential jitter was not significantly different between postsynaptic responses within the 10-pulse train ( Fig. 3b,c ). This result indicates that an alteration in the precision of spike timing is the result of modified release dynamics during trains of stimuli. 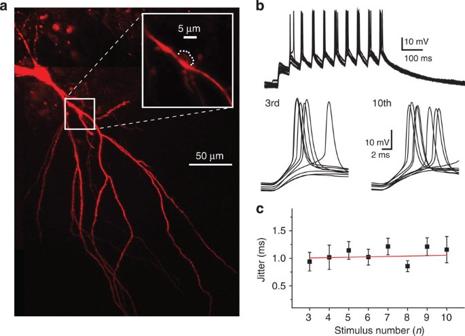Figure 3: Action potential jitter does not decrease during glutamate uncaging. (a) Example of CA3 pyramidal neuron labelled with Alexa-594. The white box indicates the apical dendritic region expanded on inset. Points of glutamate uncaging are shown as white dots around the dendritic spine. (b) Example of postsynaptic spikes evoked in this pyramidal cell by glutamate uncaging repeated at 20 Hz frequency. Action potentials evoked by the third and tenth stimuli are expanded, nine responses are shown. (c) Action potential jitter (calculated within a 8 ms window after uncaging) does not change during the train, in contrast to electrical stimulation (n=5). Red line corresponds to the linear fit of the data. Error bars show s.e.m. Figure 3: Action potential jitter does not decrease during glutamate uncaging. ( a ) Example of CA3 pyramidal neuron labelled with Alexa-594. The white box indicates the apical dendritic region expanded on inset. Points of glutamate uncaging are shown as white dots around the dendritic spine. ( b ) Example of postsynaptic spikes evoked in this pyramidal cell by glutamate uncaging repeated at 20 Hz frequency. Action potentials evoked by the third and tenth stimuli are expanded, nine responses are shown. ( c ) Action potential jitter (calculated within a 8 ms window after uncaging) does not change during the train, in contrast to electrical stimulation ( n =5). Red line corresponds to the linear fit of the data. Error bars show s.e.m. Full size image Vesicles contribute to asynchronous release Our data indicate that information transfer is altered in an activity-dependent manner and asynchronous release could potentially influence this phenomenon. However, our pharmacological approach is not suitable to determine this question since EGTA-AM had significantly altered the degree of short-term facilitation of the synchronous component. Our aim was to study the properties of information transfer under experimental conditions when asynchronous release can selectively be suppressed without influencing the properties of the synchronous component. It is known that increased synaptic activity leads to augmented vesicle recycling via the bulk endocytotic pathway [11] . Vesicle formation through this recycling pathway is dependent on the proper functioning of the AP-3. Therefore we used AP-3b2 KO animals to determine whether asynchronous release is altered in the absence of vesicles generated via the bulk endocytotic pathway. We compared the frequency of asynchronously released synaptic events between wild-type (WT) and AP-3b2 KO animals in response to short stimulus trains (10 evoked EPSCs (eEPSCs) at 20 Hz) ( Fig. 4a ). The frequency of EPSCs measured in the 500 ms time-window 200 ms after the last stimulus was almost twofold lower in AP-3b2 KOs (4.4±0.3 Hz versus 7.8±0.6 Hz; ( Fig. 4c ). In contrast, various properties of spontaneous EPSCs (sEPSCs) were similar: frequency ~3.5 Hz ( Fig. 4c ), peak amplitude~48 pA, time-to-peak ~2.7 ms and decay tau ~5 ms. Moreover, the peak amplitude of eEPSCs, as well as the degree of facilitation was not affected by the absence of AP-3b2 ( Fig. 4d ). Interestingly, the cumulative charge transferred after each stimulus starting from the second was significantly smaller in KOs ( Fig. 4e ). Furthermore, while the fast decay time constant (tau1) of the evoked response (measured at the last eEPSC) was not different between WTs and AP-3b2 KOs (8.9±0.3 ms and 8.5±0.2 ms, respectively), the slow decay time constant (tau2) and the total cumulative charge of the evoked response were significantly larger in WT mice (101.7±3.2 ms versus 89.8±3.1 ms; 152±10 pC versus 113±6 pC for WTs and KOs, respectively, Fig. 4f ). These data indicate that asynchronous release is strongly reduced in AP-3b2 KO animals possibly due to the lack of vesicles derived through AP-3-dependent endocytosis. In contrast, synchronous release is largely unaffected by the lack of AP-3. 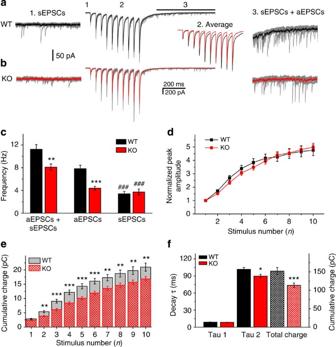Figure 4: Primary contribution of AP-3-derived vesicles to the asynchronous release. EPSCs recorded in response to 20-Hz stimulation trains (10 stimuli) in WT (a) and KO (b) mice. Ten individual responses are shown in grey, averaged evoked EPSCs in black (WT) and red (KO) are compared on the middle panel (2). Expanded regions show spontaneous (sEPSCs, left) and asynchronous (aEPSCs, right) events analyzed within 500 ms before stimulation (1) and 200 ms after stimulation (black line, 3), respectively. (c) Frequency of aEPSCs in comparison with total EPSC (aEPSCs+sEPSCs) and sEPSC frequencies. Note a significantly higher aEPSC frequency in WT mice compared with KO and similar sEPSCs frequency. In both cases sEPSC frequency was significantly lower than the total EPSC frequency after stimulation (*P<0.05, **P<0.01, ***P<0.001 and###P<0.001; Student’st-test). (d) Normalized potentiation of the synchronous component (eEPSCs) is similar between WTs and KOs, while the cumulative charge evoked by stimuli two to ten is significantly smaller in KOs (e). (f) Bar graph shows that the fast decay component (Tau1) of EPSCs evoked by the10th stimuli is not different in WTs and KOs. In contrast, the slow decay component (Tau2) and the total cumulative charge are significantly higher in WTs, due to the larger number of asynchronous EPSCs (WTn=27, KOn=33). Error bars show s.e.m. Figure 4: Primary contribution of AP-3-derived vesicles to the asynchronous release. EPSCs recorded in response to 20-Hz stimulation trains (10 stimuli) in WT ( a ) and KO ( b ) mice. Ten individual responses are shown in grey, averaged evoked EPSCs in black (WT) and red (KO) are compared on the middle panel (2). Expanded regions show spontaneous (sEPSCs, left) and asynchronous (aEPSCs, right) events analyzed within 500 ms before stimulation (1) and 200 ms after stimulation (black line, 3), respectively. ( c ) Frequency of aEPSCs in comparison with total EPSC (aEPSCs+sEPSCs) and sEPSC frequencies. Note a significantly higher aEPSC frequency in WT mice compared with KO and similar sEPSCs frequency. In both cases sEPSC frequency was significantly lower than the total EPSC frequency after stimulation (* P <0.05, ** P <0.01, *** P <0.001 and ### P <0.001; Student’s t -test). ( d ) Normalized potentiation of the synchronous component (eEPSCs) is similar between WTs and KOs, while the cumulative charge evoked by stimuli two to ten is significantly smaller in KOs ( e ). ( f ) Bar graph shows that the fast decay component (Tau1) of EPSCs evoked by the10th stimuli is not different in WTs and KOs. In contrast, the slow decay component (Tau2) and the total cumulative charge are significantly higher in WTs, due to the larger number of asynchronous EPSCs (WT n =27, KO n =33). Error bars show s.e.m. Full size image Synchronous and spontaneous release are unaltered in KOs Next, we assessed the basic parameters of mossy fibre EPSCs using quantal analysis to unequivocally demonstrate that in AP-3b2 KO animals synchronous release is not altered. We calculated the following quantal parameters: probability of release ( P ), quantal size ( Q ) and number of release sites ( N ) from EPSCs evoked with mossy fibre stimulation. It has been previously reported that mossy fibre-CA3 pyramidal cell synapses have a very low release probability even at high extracellular calcium concentration (4 mM (ref. 37 )), under these circumstances N and P cannot be reliably estimated. To overcome this problem we stimulated the presynaptic input with short trains instead of a single stimulus ( Fig. 5a ). Non-stationary variance–mean analysis of the short EPSCs trains was initially proposed and successfully used to measure quantal parameters at the Calyx of Held [38] , [39] . Only cells with stable EPSC amplitudes over 24–50 stimuli were included in the analysis ( Fig. 5b ). Variance–mean data from most of the recorded neurons were suitable for a parabolic fit (12 out of 13 neurons from WT mice and 13 out of 15 neurons from KOs) and gave the estimated value for all three quantal parameters ( Fig. 5c–e ). Quantal size ( Q ) and number of release sites ( N ) calculated from parabolic fit to the pooled data were similar in WTs and KOs (51±6 pA versus 62±6 pA, and 42±12 sites versus 30±6 sites, respectively Fig. 5c ). Moreover, none of the measured quantal parameters ( Q, N and P ) were significantly altered in the absence of AP-3b2 adaptor protein ( Fig. 5d,e ). Since bulk endocytosis is triggered in an activity-dependent manner, it may influence the rate of vesicle recycling during sustained stimulation. To investigate whether the dynamics of RRP refilling is altered in the absence of AP-3b2, we measured the size and the recovery rate of the RRP during sustained stimulation. High frequency, long-lasting stimulus (50 Hz, 60 s) was used to fully deplete the RRP ( Fig. 5f,g ). Both WTs and KOs had similar RRP size (4,404±370 vesicles, WTs; 3,915±619 vesicles, KOs), as well as number of vesicles per release sites (95±6 vesicles, WTs; 75±19 vesicles, KOs, Fig. 5h . The percentage and speed of RRP recovery were calculated using a second stimulation train delivered with a 10 s delay. There was no significant difference between the two parameters ( Fig. 5i ). 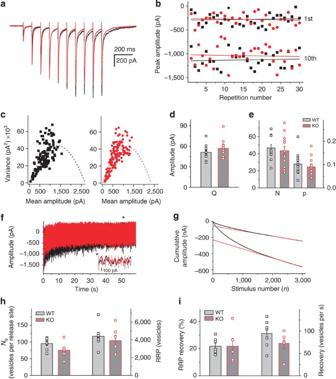Figure 5: Quantal parameters of synchronous release and the releasable vesicle pool size are not affected in AP-3 KO animals. (a) Averaged eEPSCs recorded during stimulation trains (10 Hz, 10 stimuli) in ACSF containing 4 mM [Ca2+]. (b) Peak amplitudes of the 1st and 10th eEPSCs in a train are plotted against repetition number and fitted with linear fit, solid-black (WT) and red (KO) lines to exclude the involvement of long-term plastic changes. (c) Pooled variance–mean plots and parabolic fits are shown as dashed lines (WT—black,n=13 and KO—red,n=15). (d) Comparison of calculated quantal sizeQin WTs,n=13 and KOs,n=15. (e) Number of release sites (N) and initial release probability (P) calculated from parabolic fits (WTn=12, KOn=13). Data for individual cells are shown as black squares (WT) and red circles (KO). None of the parameters are significantly different. (f) eEPSCs amplitude during stimulation train (50 Hz, 3,000 stimuli), black and response to the same stimulation 10 s later, red. Note a smaller amplitude of the response to the second train. Inset shows expanded response at the end of the train (*) after vesicle depletion. Corresponding cumulative amplitudes are shown ing. Dashed lines represent back extrapolated linear fits obtained from last 1,000 stimuli (solid red). WT data are shown. (h,i) Comparison of the number of vesicles per release site (Nq, WTn=8, KOn=6), size of ready releasable pool of vesicles (RRP), percentage and speed of RRP recovery after 10 s (WTn=9, KOn=6). The data for individual cells are shown as black squares (WT) and red circles (KO). Error bars show s.e.m. Figure 5: Quantal parameters of synchronous release and the releasable vesicle pool size are not affected in AP-3 KO animals. ( a ) Averaged eEPSCs recorded during stimulation trains (10 Hz, 10 stimuli) in ACSF containing 4 mM [Ca 2+ ]. ( b ) Peak amplitudes of the 1st and 10th eEPSCs in a train are plotted against repetition number and fitted with linear fit, solid-black (WT) and red (KO) lines to exclude the involvement of long-term plastic changes. ( c ) Pooled variance–mean plots and parabolic fits are shown as dashed lines (WT—black, n =13 and KO—red, n =15). ( d ) Comparison of calculated quantal size Q in WTs, n =13 and KOs, n =15. ( e ) Number of release sites ( N ) and initial release probability ( P ) calculated from parabolic fits (WT n =12, KO n =13). Data for individual cells are shown as black squares (WT) and red circles (KO). None of the parameters are significantly different. ( f ) eEPSCs amplitude during stimulation train (50 Hz, 3,000 stimuli), black and response to the same stimulation 10 s later, red. Note a smaller amplitude of the response to the second train. Inset shows expanded response at the end of the train (*) after vesicle depletion. Corresponding cumulative amplitudes are shown in g . Dashed lines represent back extrapolated linear fits obtained from last 1,000 stimuli (solid red). WT data are shown. ( h , i ) Comparison of the number of vesicles per release site ( N q, WT n =8, KO n =6), size of ready releasable pool of vesicles (RRP), percentage and speed of RRP recovery after 10 s (WT n =9, KO n =6). The data for individual cells are shown as black squares (WT) and red circles (KO). Error bars show s.e.m. Full size image Short-term synaptic plasticity is influenced by several pre and postsynaptic factors, among those temporal properties of neurotransmitter release is frequently assessed as paired pulse ratio (PPR) [40] . We calculated PPR of two stimuli at 20 Hz, delivered at 0.1–5 Hz basal frequency and did not observe any difference between the amplitudes of the evoked events in WTs and AP-3b2 KOs ( Fig. 6a,b ). Next, we compared EPSC responses to longer trains. Twenty responses were recorded at each stimulation frequency ( Fig. 6c ). Prominent short-term facilitation was observed both in WTs and AP-3b2 KOs, and the degree of facilitation was not different between groups. A small difference in EPSC amplitude was detected at 0.5 and 5 Hz, but this was not consistently observed in the normalized data ( Fig. 6d,e ). At all tested stimulation frequencies, kinetic properties—such as time-to-peak and decay time constant—were not different ( Fig. 6f,g ). These data suggest that prominent short-term facilitation can be supported in the absence of vesicles derived through bulk endocytosis. 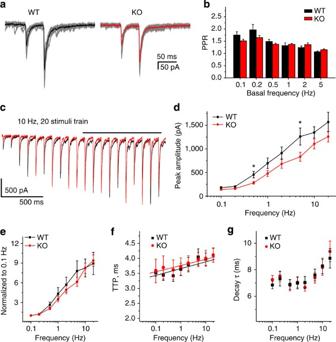Figure 6: Short-term plasticity is not altered by AP-3 deletion. (a) EPSCs evoked using paired pulse stimulation protocol. Individual responses are shown in grey; black and red traces correspond to the averaged responses for WT and KO, respectively. (b) Paired pulse ratio calculated at different basal frequencies (paired pulse was given at 20 Hz). (c) Example of averaged responses for WTs (black) and KOs (red) evoked by 10-Hz stimulation train. Peak amplitude and kinetic properties were measured after potentiation reached plateau (last 10 EPSCs, solid-black line). Graphs are depicting the correlation between averaged peak amplitude (d), normalized peak amplitude (e), TTP (f), decay time constant (g) and the stimulation frequency. The level of short-term plasticity in KO (n=9, red) animals compared with WTs (n=7, black) is similar (except for the 0.5 and 5 Hz) before normalization (d). At all tested frequencies, TTP and decay time constant are not significantly different. Solid lines correspond to the linear fits (f). *P<0.05; Student’st-test. Error bars show s.e.m. Figure 6: Short-term plasticity is not altered by AP-3 deletion. ( a ) EPSCs evoked using paired pulse stimulation protocol. Individual responses are shown in grey; black and red traces correspond to the averaged responses for WT and KO, respectively. ( b ) Paired pulse ratio calculated at different basal frequencies (paired pulse was given at 20 Hz). ( c ) Example of averaged responses for WTs (black) and KOs (red) evoked by 10-Hz stimulation train. Peak amplitude and kinetic properties were measured after potentiation reached plateau (last 10 EPSCs, solid-black line). Graphs are depicting the correlation between averaged peak amplitude ( d ), normalized peak amplitude ( e ), TTP ( f ), decay time constant ( g ) and the stimulation frequency. The level of short-term plasticity in KO ( n =9, red) animals compared with WTs ( n =7, black) is similar (except for the 0.5 and 5 Hz) before normalization ( d ). At all tested frequencies, TTP and decay time constant are not significantly different. Solid lines correspond to the linear fits ( f ). * P <0.05; Student’s t -test. Error bars show s.e.m. Full size image Previously, spontaneous neurotransmitter release has been shown to regulate postsynaptic excitability and spike timing [41] , [42] . Therefore, we compared the frequency and kinetic properties of mEPSCs recorded from CA3 pyramidal cells in the presence of 1 μM tetrodotoxin (TTX) between WT and KO animals. We did not find any significant difference between the parameters we investigated: for WTs and KOs average frequency: 0.97±0.2 Hz and 1.09±0.18 Hz, peak amplitude: 42±1 pA and 49±1 pA, time-to-peak: 2.75±0.02 ms and 2.79±0.02 ms and decay time constant: 4.86±0.08 ms and 5.08±0.06 ms, respectively. To determine whether these physiological differences observed in AP-3b2 KOs could be correlated with morphological alterations, we investigated the distribution of vesicles in mossy fibre synapses from WT and KO mice using electron microscopy ( Supplementary Fig. 3A ). Total vesicle density, the number of docked vesicles and vesicle density at various distances from active zone was not significantly different between WTs and KOs ( Supplementary Fig. 3B ). These results suggest that vesicles contributing to various forms of releases are not segregated to distinct compartments of the presynaptic terminal. Diminished asynchronous release during trains in KOs To investigate the change in the asynchronous release rate during stimulation trains, we conducted experiments with stimulation at 20 Hz frequency while increasing number of stimuli from 2 to 8 ( Fig. 7a–d ). aEPSCs were analyzed at the same time-window as after 10-stimuli trains ( Figs 2 and 4 ). In WTs, the increase in the number of stimuli resulted in the linear rise of asynchronous release, measured as frequency of aEPSCs, from 2.3±0.8 to 9.5±1.3 Hz ( Fig. 7e ). Interestingly, in KOs this rise of asynchronous release was significantly impaired starting already from two stimuli and was two times smaller after eight stimuli (4.2±1 Hz, Fig. 7e ). 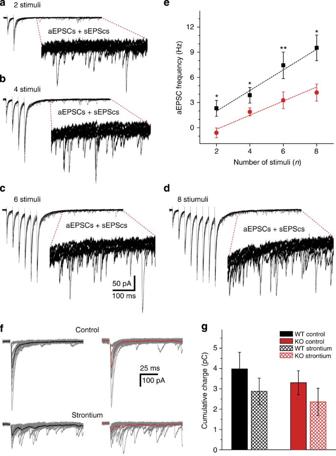Figure 7: Asynchronous release increases with the number of stimuli and impaired in AP-3 KOs. aEPSCs after, 2 (a), 4 (b), 6 (c) and 8 (d) stimuli delivered at 20 Hz, 15 sweeps are shown. Inserts show expanded 500 ms regions with a mixture of aEPSCs and sEPSCs. (e) Average data showing increase in the aEPSCs frequency with the number of stimuli. This increase was significantly smaller in KOs (n=7) compared with WTs (n=7). Dashed lines correspond to the linear fits. (f) eEPSCs recorded at 0.5 Hz frequency in control conditions (top) and in the presence of 6 mM strontium (bottom) in WT (left) and KO (right) mice. Fifteen individual traces are shown in grey, averaged eEPSCs are shown in black and red (f). (g) Bar graph showing that total cumulative charge is not significantly different between WTs (n=7) and KOs (n=6) in control conditions (P=0.53) and after strontium application (P=0.59). *P<0.05 and **P<0.01; Student’st-test. Error bars show s.e.m. Figure 7: Asynchronous release increases with the number of stimuli and impaired in AP-3 KOs. aEPSCs after, 2 ( a ), 4 ( b ), 6 ( c ) and 8 ( d ) stimuli delivered at 20 Hz, 15 sweeps are shown. Inserts show expanded 500 ms regions with a mixture of aEPSCs and sEPSCs. ( e ) Average data showing increase in the aEPSCs frequency with the number of stimuli. This increase was significantly smaller in KOs ( n =7) compared with WTs ( n =7). Dashed lines correspond to the linear fits. ( f ) eEPSCs recorded at 0.5 Hz frequency in control conditions (top) and in the presence of 6 mM strontium (bottom) in WT (left) and KO (right) mice. Fifteen individual traces are shown in grey, averaged eEPSCs are shown in black and red ( f ). ( g ) Bar graph showing that total cumulative charge is not significantly different between WTs ( n =7) and KOs ( n =6) in control conditions ( P =0.53) and after strontium application ( P =0.59). * P <0.05 and ** P <0.01; Student’s t -test. Error bars show s.e.m. Full size image Various properties of asynchronous release are often assessed in the presence of strontium. The replacement of calcium with strontium leads to the desynchronization of the evoked response. In our previous experiments, we found selective deficits in asynchronous release in AP-3b2 KOs; we decided to determine whether similar differences could be observed in the presence of strontium. Towards this aim, we recorded evoked mossy fibre EPSCs in ACSF containing: 6 mM SrCl 2 /0 mM CaCl 2 /0 mM MgCl 2 . This substitution resulted in prominent EPSC desynchronization in both genotypes ( Fig. 7f ). However there was no significant difference in the transferred cumulative charge between WTs and AP-3b2 KOs ( Fig. 7g ). These results suggest that the surrogate strontium leads to the desynchronization of the entire vesicle pool: the time course of the fusion of vesicles contributing to synchronous and asynchronous release is indistinguishable. Conversely, in normal ASCF the differential temporal release dynamics of the asynchronous component enables the separate detection and analysis of these events. Neurotransmitter release rate can be assessed directly by the deconvolution method from recorded EPSCs using Fourier transform ( Fig. 8a,b ). We used this approach to determine the time course of neurotransmitter release during stimulation trains. This approach allows us to determine changes in the ratio of synchronous and asynchronous release. To distinguish between the two modes of neurotransmitter release we separately calculated the cumulative rate of synchronous and asynchronous release in response to each stimulus ( Fig. 8c,d ). Synchronous release was measured in the first 10 ms following each stimuli; the values were not significantly different between WTs and AP-3b2 KOs ( Fig. 8d ). After the third response KO animals had a significantly reduced rate of asynchronous release, approximately half of the rate observed in WTs ( Fig. 8e ). Although the asynchronous release rate is much smaller than the synchronous component ( Fig. 8d,e ) this diminution effectively reduced the total neurotransmitter release rate (36.8±2.7 quanta per s and 27.3±2.5 quanta per s, respectively, for WT and KO mice, P =0.028, Fig. 8f ). To investigate the correlation between the two forms of release and AP jitter, the measurements of synchronous and asynchronous release components obtained using a deconvolution method ( Fig. 8d,e ) were plotted together with the AP jitter (data from Fig. 2e ) as a function of stimulus number ( Fig. 8g ). This plot clearly shows that the largest change in AP jitter occurs when synchronous release reaches a steady-state phase in contrast to the asynchronous release that continues to rise rapidly. 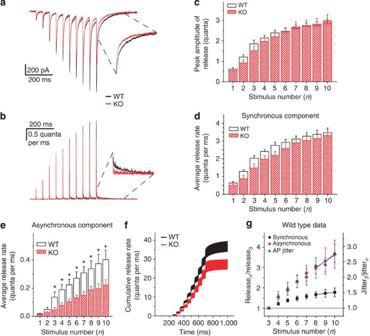Figure 8: Deconvolution analysis of evoked EPSCs. (a) Averaged EPSCs evoked by stimulation trains (20 Hz, 10 stimuli) and the corresponding release rate (b) are calculated using the deconvolution method. Inserts are showing expanded regions; note the difference in decay between WTs and KOs. (c) Quantified release rate: The peak amplitude of release (c) and synchronous rate (integrated within the first 10 ms following each stimulus) (d) are similar in response to all 10 stimuli. Asynchronous rate of release (integrated between 10 and 50 ms after each stimulus) (e) is significantly higher in WTs, starting from the third response. Reduced asynchronous release significantly affects the total cumulative release (f). WTn=7, KOn=6. (g) Deconvolution data shown together with AP jitter from separate sets of cells. Note that by the end of train the synchronous release (black) increase reaches a plateau; while increases in asynchronous release (red) and AP jitter (blue) continue to rise. Data are normalized to the third response. Solid lines correspond to linear fits. *P<0.05; Student’st-test. Error bars show s.e.m. Figure 8: Deconvolution analysis of evoked EPSCs. ( a ) Averaged EPSCs evoked by stimulation trains (20 Hz, 10 stimuli) and the corresponding release rate ( b ) are calculated using the deconvolution method. Inserts are showing expanded regions; note the difference in decay between WTs and KOs. ( c ) Quantified release rate: The peak amplitude of release ( c ) and synchronous rate (integrated within the first 10 ms following each stimulus) ( d ) are similar in response to all 10 stimuli. Asynchronous rate of release (integrated between 10 and 50 ms after each stimulus) ( e ) is significantly higher in WTs, starting from the third response. Reduced asynchronous release significantly affects the total cumulative release ( f ). WT n =7, KO n =6. ( g ) Deconvolution data shown together with AP jitter from separate sets of cells. Note that by the end of train the synchronous release (black) increase reaches a plateau; while increases in asynchronous release (red) and AP jitter (blue) continue to rise. Data are normalized to the third response. Solid lines correspond to linear fits. * P <0.05; Student’s t -test. Error bars show s.e.m. Full size image Asynchronous release influences action potential jitter Action potential probability and timing are two key parameters of synaptic information processing. We compared these parameters between WT and AP-3b2 KO animals to determine whether asynchronous release has any significant influence on these measures. We used in vivo stimulus patterns to stimulate mossy fibres ( Fig. 9a ) and calculated action potential probability from postsynaptic signal recordings of CA3 pyramidal cells. We only observed significant differences in the probability of postsynaptic spike generation between WTs and KOs in response to the small fraction of the stimuli (8–19%, Fig. 9b ). In contrast, the activity-dependent increase in the precision of spike timing was largely eliminated in AP-3b2 KO animals ( Fig. 9c–e ). Moreover, during 20 Hz train stimulation in KOs, AP jitter did not reduce significantly by the end of the train ( Fig. 9f ) and was larger compared with WTs ( Fig. 9g ). These results suggest that vesicles derived through the AP-3-dependent recycling pathway play a role in the regulation of action potential timing during increased presynaptic activity. 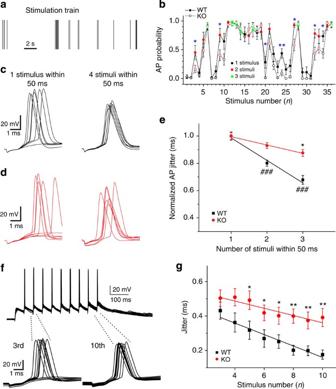Figure 9: Action potential dejittering is impaired in AP-3b2 KO mice. (a) Example of a natural stimulation train and the corresponding probability of evoked postsynaptic action potentials (b). Responses to small number of stimuli were different in WTs and KOs (5 out of 36). Examples of evoked postsynaptic spikes recorded in WTs (c) and KOs (d), seven responses are shown. Note that the difference in action potential jitter between single stimulation (one stimulus within 50 ms, left) and burst stimulation (three stimuli within 50 ms, right) is not present in KOs. (e) Plot showing normalized action potential jitter as a function of the number of stimuli within 50 ms in WTs (black,n=18) and KOs (red,n=19). In contrast to WTs, action potential jitter does not change with the frequency of the presynaptic stimulus in KOs and is significantly larger after short burst stimulation. Dashed lines indicate an example of corresponding stimulus number inb, stimuli were grouped into categories 1 and 3. (f) Example of postsynaptic APs evoked by 10 stimuli at 20 Hz in KO mice. APs evoked by the 3rd and 10th stimuli are expanded, 10 responses are shown. Note the similar AP jitter at the beginning and end of the train. (g) Average plot showing that AP jitter calculated within 6 ms after stimulation is significantly larger in KOs (n=13) compared with WTs (n=7), and does not decrease significantly during train stimulation. *P<0.05, **P<0.01 and###P<0.001; Student’st-test. Error bars show s.e.m. Figure 9: Action potential dejittering is impaired in AP-3b2 KO mice. ( a ) Example of a natural stimulation train and the corresponding probability of evoked postsynaptic action potentials ( b ). Responses to small number of stimuli were different in WTs and KOs (5 out of 36). Examples of evoked postsynaptic spikes recorded in WTs ( c ) and KOs ( d ), seven responses are shown. Note that the difference in action potential jitter between single stimulation (one stimulus within 50 ms, left) and burst stimulation (three stimuli within 50 ms, right) is not present in KOs. ( e ) Plot showing normalized action potential jitter as a function of the number of stimuli within 50 ms in WTs (black, n =18) and KOs (red, n =19). In contrast to WTs, action potential jitter does not change with the frequency of the presynaptic stimulus in KOs and is significantly larger after short burst stimulation. Dashed lines indicate an example of corresponding stimulus number in b , stimuli were grouped into categories 1 and 3. ( f ) Example of postsynaptic APs evoked by 10 stimuli at 20 Hz in KO mice. APs evoked by the 3rd and 10th stimuli are expanded, 10 responses are shown. Note the similar AP jitter at the beginning and end of the train. ( g ) Average plot showing that AP jitter calculated within 6 ms after stimulation is significantly larger in KOs ( n =13) compared with WTs ( n =7), and does not decrease significantly during train stimulation. * P <0.05, ** P <0.01 and ### P <0.001; Student’s t -test. Error bars show s.e.m. Full size image One of the possible mechanisms by which asynchronous release is able to affect action potential precision is by providing additional slow depolarization. This depolarization can accumulate during repetitive activity due to the increasing number of asynchronously released vesicles. Indeed, the analysis of current-clamp recordings revealed that on an average slow depolarization was 4 mV smaller by the end of a 10-stimuli train in KOs compared with WTs. To test whether this slow depolarization could affect action potential jitter we added ramp depolarization starting after the 2nd stimuli and rising to 4 mV by the 10th stimuli in KOs ( Supplementary Fig. 4 ). The amount of injected current, sufficient to raise the membrane voltage by 4 mV, was determined for each recorded neuron and varied from 30 to 50 pA ( Supplementary Fig. 4A ). Repetitive stimulation in current-clamp mode evoked action potentials with high jitter even at the end of the 10-stimuli train ( Supplementary Fig. 4B ), however spiking precision was significantly improved by application of ramp depolarization ( Supplementary Fig. 4B,C ). These results indicate that slow depolarization provided by asynchronously released vesicles are essential for the regulation of action potential precision at mossy fibre–CA3 pyramidal cell synapses. Asynchronous release alters information transfer The amplitude and the temporal properties of the incoming signal influence synaptic information transfer. While our data showed that asynchronous release does not significantly alter short-term plasticity we also found that, in the absence of vesicles contributing to asynchronous release, activity-dependent decrease in action potential jitter is absent during increased activity. Next, we aimed to investigate how global information transfer is influenced by the deficit in asynchronous release during natural stimuli patterns. We chose four different stimulus patterns from in vivo granule cell firing patterns containing bursts embedded into low frequency activity (all chosen patterns were recorded during left–right alternation task from three different animals). In each stimulus pattern, the ratio of action potentials occurring under conditions when asynchronous release could be triggered was different. Since we found that asynchronous release becomes significant after the third stimulus in a train, we identified regions as ‘asynchronous release friendly’ when action potentials were preceded by at least two stimuli and occurred at 10–100 Hz. The ratio varied between 11 and 22% in the four-stimulus trains ( Fig. 10a ). To investigate information transfer we calculated SR and RR coherences using binary representation of recorded responses ( Fig. 10b,c ), as described in the Methods. The difference between the square root of RR coherence and SR coherence corresponds to the theoretically possible amount of encoded information. There was no significant difference in the RR coherence calculated separately for each stimulation train ( Fig. 10b–d ). The transferred information was significantly lower in reduced asynchronous release conditions, in response to the first stimulation train (1.96±0.08, n =8 for WTs and 1.68±0.05, n =10 for KOs) ( Fig. 10e ). Moreover, the difference in the calculated information between WTs and AP-3b2 KOs showed a linear correlation with the percentage of spikes occurring under conditions where asynchronous release can occur ( Fig. 10f ). These results suggest that under certain conditions asynchronous release could be essential for reliable information transfer between granule cells and pyramidal cells, and could significantly contribute to neuronal coding. 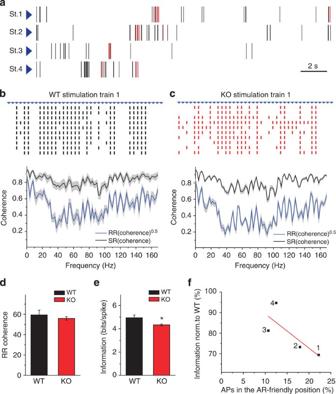Figure 10: Impaired information transfer during natural-like stimulation patterns due to reduced asynchronous release. (a) Four stimulation trains used in the experiments. Action potentials occurring under conditions when asynchronous release can be evoked are highlighted in red (22%, 18%, 12.5% and 11% of total stimulus number for stimulation trains 1, 2, 3 and 4 respectively). (b) An example of postsynaptic responses (action potentials) evoked by the first stimulation train (St. 1;a) in WT (b, top) and KO (c, top) cells. Data are presented in binary format, 10 consecutive trials are shown. Averaged square rooted RR coherence and SR coherence calculated for responses to the St. 1 in WTs (b, bottomn=8) and KOs (c, bottomn=10). Integrated from 0 to 168 Hz RR coherence (d) and transferred information per spike (e). Information in response to the first stimulation train is significantly smaller in KOs, while coherence is similar. (f) Difference in the total transferred information between WTs and KOs dependent on the percentage of action potentials occurring in asynchronous release friendly positions (see text for definition). Four points correspond to four different stimulation trains. Solid line corresponds to linear fit of the data. Total 19 WT neurons and 25 KO neurons were stimulated with 1–3 different stimulation patterns. *P<0.05; Student’st-test. Error bars show s.e.m. Figure 10: Impaired information transfer during natural-like stimulation patterns due to reduced asynchronous release. ( a ) Four stimulation trains used in the experiments. Action potentials occurring under conditions when asynchronous release can be evoked are highlighted in red (22%, 18%, 12.5% and 11% of total stimulus number for stimulation trains 1, 2, 3 and 4 respectively). ( b ) An example of postsynaptic responses (action potentials) evoked by the first stimulation train (St. 1; a ) in WT ( b , top) and KO ( c , top) cells. Data are presented in binary format, 10 consecutive trials are shown. Averaged square rooted RR coherence and SR coherence calculated for responses to the St. 1 in WTs ( b , bottom n =8) and KOs ( c , bottom n =10). Integrated from 0 to 168 Hz RR coherence ( d ) and transferred information per spike ( e ). Information in response to the first stimulation train is significantly smaller in KOs, while coherence is similar. ( f ) Difference in the total transferred information between WTs and KOs dependent on the percentage of action potentials occurring in asynchronous release friendly positions (see text for definition). Four points correspond to four different stimulation trains. Solid line corresponds to linear fit of the data. Total 19 WT neurons and 25 KO neurons were stimulated with 1–3 different stimulation patterns. * P <0.05; Student’s t -test. Error bars show s.e.m. Full size image Prominent asynchronous release has been described in both excitatory and inhibitory synaptic connections [7] , [33] , [43] , [44] , [45] . Asynchronous GABA release from hippocampal interneurons is responsible for the switch from phasic to the prolonged inhibition exhibited during periods of increased activity [45] , [46] . The importance of asynchronous release in synchronization was defined at the cerebellum: synapses from deep cerebellar nuclei to the inferior olive neurons release GABA almost exclusively in an asynchronous manner [6] , which resulted in steady-state inhibition during high frequency activity. This persistent inhibitory current not only suppressed inferior olive neurons firing, but also reduced the effectiveness of their electrical coupling, leading to desynchronization. Manseau et al. [47] had shown that asynchronous GABA release from fast spiking somatosensory neurons is able to desynchronize local networks and interfere with information processing in the cortex. Asynchronous glutamate release from the cerebellar granule cells is prominent in response to individual presynaptic action potentials. It can become comparable to synchronous release in response to short action potential bursts [33] . The authors proposed that this could serve as a form of short-term memory mechanism, preserving information about the history of neuronal activity. This seems to be true for paraventricular nucleus magnocellular neurons exhibiting asynchronous glutamate release in response to burst stimulation, which results in prolonged postsynaptic spiking [7] . At these synaptic connections, asynchronous release may help to integrate several inputs from different nuclei over time, ensuring reliable information transfer during high activity levels. It was shown in hippocampal cultures that asynchronous glutamate release plays a central role in the reverberatory activity of the network and might be important for working memory. Our data support the important role of asynchronous release in information transfer and processing. We analyzed two important parameters of neuronal coding SR and RR coherences, both of them varying between 0 and 1, reporting on different physiological properties. RR coherence is calculated from repetitive presentation of the stimulation pattern to the same neuron and measures the strength to which the responses are correlated at a given frequency [48] , [49] . Thus, RR coherence characterizes the reproducibility of synaptic responses to a particular stimulation pattern, where higher RR coherence corresponds to more consistent responses. The absence of difference in RR coherence between WTs and KOs suggests that upper limit for transmitted information was not altered. In contrast, SR coherence is calculated for a particular stimulation pattern and estimates how closely various stimulation frequencies are represented by the output firing of neurons [48] , [50] . SR coherence was used to calculate total transferred information and information per single postsynaptic spike, as describe in the Methods. We observed a significant reduction of the transferred information in response to certain natural stimulation patterns when asynchronous release was decreased. Based on the properties of asynchronous release we suggest that information transmission at gamma range frequencies (20–100 Hz) should be most dependent on asynchronous release. At higher frequencies the summation of synchronous EPCSs would be sufficient to trigger reliable action potentials, whereas at lower frequencies, asynchronous release would decay before the arrival of the next stimulus. This idea is indirectly supported by our data on the postsynaptic spike synchronization. The presence of at least one preceding stimuli within 50 ms (≥20 Hz, between stimuli) significantly reduces action potential jitter due to the action of asynchronous release, and this effect is absent in KO animals. We suggest that asynchronous glutamate release from mossy fibre boutons plays a major role in information coding by increasing the reliability of information transfer and enhancing its temporal precision. Similarly to asynchronous release, activation of postsynaptic kainate receptors during short trains leads to the development of sustained depolarization [51] , and presynaptic kainate receptors have been shown to contribute to short-term facilitation at mossy fibre synapses [52] , [53] , [54] (but see the study by Kwon et al. [55] ). The contribution of kainate receptors to the difference we observed between WT and Ap-3b2 KO animals is unlikely for the following reasons: presynaptic kainate receptors significantly alter short-term plasticity at mossy fibre synapses, and we did not observe any change in the facilitation of the synchronous component in Ap-3b2 KO animals, suggesting that presynaptic kainate receptor function is unaltered. In addition, attenuated postsynaptic kainate receptors function is also unlikely since AP-3 is expressed in presynaptic axonal compartments [56] . Our data indicate that vesicles generated via bulk endocytosis primarily contribute to asynchronous release: in their absence information transfer is compromised, leading to less reliable neuronal coding. These findings are consistent with previous reports suggesting that distinct vesicle pools fulfil different physiological functions at the synapse. Bulk endocytosis and clathrin-dependent endocytosis has been shown to be activated under different circumstances and replenish distinct vesicle pools [21] . Vesicle recycling via intermediate endosomes relies on the proper functioning of AP-3, and the recruitment of several vesicle membrane proteins is tightly linked to this adaptor protein. The initial recruitment of AP-3, in the vesicles generated from endosomes after bulk endocytosis, could provide a reliable mechanism for the generation of a functionally heterogeneous vesicle pool. VAMP7-containing vesicles have been shown to preferentially replenish the resting pool that contributes only minimally to evoked release [23] . This particular form of v-SNARE is present at a high concentration in mossy fibre terminals, however in the mocha -mutant mice lacking AP-3, the expression is completely abolished [12] . VAMP7 is a tetanus-insensitive v-SNARE, and tetanus-toxin insensitive release is compromised in these animals [12] . Similar to VAMP7, ZnT3 and CIC3 have also been shown to be selectively present in vesicles derived through an AP-3-dependent mechanism. These findings, with our current study, suggest that vesicles recycled via bulk endocytosis and derived from endosomes through AP-3-dependent mechanisms have a unique molecular composition that preferentially targets a vesicle pool primarily contributing to asynchronous release. However, a notable difference between our current findings and results presented in the study by Huaz et al. [23] is the lack of effect on spontaneous release in our study. A contrast in spontaneous activity levels observed in cell cultures and slices could be behind this apparent discrepancy. Functionally distinct vesicle pools composed of vesicles with varying release rates were described at the Calyx of Held. Fast vesicles participated mainly in synchronous release. and slow releasing vesicles (reluctantly releasable pool) contributed to asynchronous release [9] , [57] , [58] . Our data support the idea of a heterogeneous releasable pool of vesicles. Moreover we can further specify that vesicular pools participating in the synchronous and asynchronous modes of release also preferentially recycle through different endocytotic pathways. Together these findings suggest that the heterogeneity of releasable vesicles could be a common feature of various types of synapses. Importantly, this heterogeneity is present on multiples levels: mode of release, recycling pathways and molecular composition. Thus, the slowly releasable pool of vesicles would mainly contribute to asynchronous release and recycle through bulk endocytosis followed by AP-3-dependent vesicle formation from endosomes. In contrast, the RRP of vesicles supports synchronous release and its recycling is AP-3 independent. Our data suggest that asynchronous and synchronous glutamate release utilize distinct vesicle pools. Several laboratories have addressed this question previously without reaching an obvious consensus. The competitions between the two pools have been assessed by EGTA-AM application. In hippocampal cell cultures, EGTA-AM has decreased asynchronous release while synchronous release was increased. This suggests that by eliminating asynchronous release the synchronous component can utilize a larger pool [27] . However, in our experiments EGTA-AM has decreased asynchronous release and limited short-term facilitation similar to data obtained from the cerebellar slices [33] . In other studies, EGTA-AM has selectively reduced asynchronous release without influencing the synchronous component [7] , [43] . These widely varied observations in asynchronous release and short-term plasticity with the usage of EGTA-AM could be explained with the independent action of this calcium chelator on asynchronous release and short-term plasticity. This scenario is supported by our findings where EGTA-AM application altered short-term facilitation; while in AP-3b2 KO animals, showing significantly diminished asynchronous release, short-term facilitation was unaltered. Our results support the idea that functionally distinct vesicles co-exist in the presynaptic terminal. In Ap-3b2−/− animals, vesicle density and the number of docked vesicles did not change, suggesting that in the absence of the endosomal recycling pathway other recycling pathways compensate for vesicle recycling [13] . These compensatory mechanisms increase the number of vesicles belonging to other functional pools in Ap-3b2−/− animals. The physiological consequences of this subtle increase in the number of vesicles, supporting other forms of release, are yet to be elucidated. Synchronous neurotransmitter release is regulated by the v-SNARE VAMP2 and the calcium sensors synaptotagmin 1, 2 and 9 (refs 30 , 59 , 60 ). Recently, several presynaptic proteins have been identified as specific contributors to asynchronous release. At inhibitory terminals, VAMP4 and synapsyn II have been shown to play a key role in asynchronous release [25] , [61] . Doc2 and synaptotagmin 7 are calcium sensors with activities selectively linked to asynchronous release [26] , [62] , [63] . However, the selective role of these calcium sensors in asynchronous release at central nervous system synapses is currently debated [64] , [65] , [66] . While it is tempting to speculate that selective calcium sensors regulating asynchronous release are recruited only to vesicles generated via bulk endocytosis, the relationship between various forms of calcium sensors are too complicated to reach this simplistic conclusion [67] . However, our study further highlights the functional importance of vesicular heterogeneity, which starts with their preferential release in one of the different modes (synchronous, asynchronous and spontaneous) and continues through the entire vesicular life cycle, including different routes of endocytosis and segregation into distinct vesicular pools. Acute slice preparation Hippocampal slices were prepared from AP-3b2 WT or knockout mice [31] (P17–25). All protocols were approved by the Animal Protection Committee of Université Laval. Ap-3b2 −/− animals were originally produced by the laboratory of Victor Faundez [31] . Ap-3b2−/− animals were generated by directly targeting in C57BL/6 and continued breeding on the same background. Animals were backcrossed by mating C57BL/6 animals with Ap-3b2 +/− mice. Heterozygous animals were identified by genotyping. Ap-3b2 −/− animals used in our experiments were obtained by mating heterozygous females with homozygous males. For preparation of acute hippocampal slices (300 μm), mice were anesthetized with isoflurane. Following decapitation, the brain was promptly removed from the skull and immersed in ice-cold ACSF containing : NaCl 87 mM, NaHCO 3 25 mM, KCl 2.5 mM, NaH 2 PO4 1.25 mM, MgCl 2 7 mM, CaCl 2 0.5 mM, glucose 25 mM and sucrose 75 mM. The brain was dissected and hippocampal slices were cut at an angle to optimize preservation of mossy fibres using a vibrating-blade microtome (Leica, Germany). Right after sectioning, slices were placed in oxygenated ACSF at 32 °C for 40 min, and maintained at room temperature prior to experiments. All recordings were performed with extracellular ACSF containing: NaCl 124 mM, NaHCO 3 25 mM, KCl 2.5 mM, MgCl 2 1.5 mM, CaCl 2 2.5 mM and glucose 10 mM, unless specified differently; equilibrated with 95% O 2 –5% CO 2 , pH7.4, maintained at 30–33 °C and perfused at a rate of 2–3 ml min −1 . Bicuculline methiodide (1 μM) was always present in extracellular ACSF during recordings. Electrophysiology Whole-cell current clamp and voltage-clamp recordings were made with glass electrodes (4–6.5 MΩ) filled with a solution containing: K-gluconate 120 mM, KCl 20 mM, MgCl2 2 mM, EGTA 0.6 mM, MgATP 2 mM, NaGTP 0.3 mM, Hepes 10 mM, phosphocreatine 7 mM or Cs-gluconate 100 mM, NaCl 8 mM, MgCl2 5 mM, EGTA 0.6 mM, MgATP 2 mM, NaGTP 0.3 mM, Hepes 40 mM, phosphocreatine 7 mM and QX-314 1 mM (Cs-gluconate-based solution was used for short-term plasticity experiments). Recordings were made from visually identified CA3 pyramidal neurons using a Multi Clamp 700A amplifier (Axon Instruments, Union City, CA, USA), operating under current-clamp and voltage-clamp mode. Data were filtered at 4 kHz, and acquired using pClamp 10 software (Molecular devices, Sunnyvale, CA, USA). Mossy fibre inputs were electrically stimulated via a patch micropipette placed in the stratum lucidum and identified based on their kinetic properties and profound short-term facilitation. At the end of each experiment, (2S,1′R,2′R,3′R)-2-(2,3-dicarboxycyclopropyl)-glycine (DCG-4) was applied to confirm the mossy fibre origin of the synaptic input. Recordings were done at a holding potential: −70 mV (voltage clamp) and −60 mV (current clamp). The uncompensated series resistance was monitored by the delivery of −10 mV steps throughout the experiment, only recordings with <15% change were analyzed. Drugs Hundred micromolar EGTA-AM (Anaspec, Fremont, CA, USA), 1 μM TTX (Alomone labs, Jerusalem, Israel), 1 μM DCG-4 (Tocris Bioscience, Ellisville, MO, USA), 1 μM bicuculline methiodide (Sigma-Aldrich, Canada) and 6 mM SrCl 2 (Sigma-Aldrich) were dissolved in extracellular ACSF and applied through the perfusion system (at least 5 mins before recordings). All reagents were prepared as stock solutions and stored as recommended. EGTA-AM was dissolved in properly oxygenated solution at pH 7.4. Two-photon glutamate uncaging Ultrafast two-photon glutamate uncaging was performed with a two-photon imaging system (Kaluti System, France) equipped with acousto-optic deflectors (AODs, A–A Opto-Electronics, France) and connected to a Ti-Sapphire pulsed laser (Chameleon Ultra, repetition rate=80 MHz, pulse width=140 fs, power >3.5 W, Coherent, CA, USA) tuned at 720 or 800 nm. AODs allowed for fast non-mechanical laser beam movement in the x - and y -dimensions. The laser was focused with a high numerical aperture water-immersion Leica × 25 objective (numerical aperture=0.95) under an upright microscope. The imaging system and laser were controlled with custom-made software written in Labview [27] . Individual CA3 pyramidal cells were identified and targeted for patch-clamp recordings with a DODT scanning-gradient contrast. Whole-cell current-clamp recordings were obtained from CA3 pyramidal cells with potassium-based patch solution supplemented with 40 μM Alexa-594 (Life Technologies, CA, USA). Cells were passively filled with the fluorescent molecule for 10 min before starting the experiments. To inspect the morphology of the neuron, the morphological dye was excited at 800 nm and emitted photons were collected in the trans-fluorescence configuration through an oil condenser (numerical aperture=1.4). Photons were band-pass filtered at 580–667 nm (Semrock, NY, USA) and detected with a cooled AsGaP Hamamatsu (H7422P-40) photomultiplier tube. Thorny excrescences were identified on the apical dendritic trunk of CA3 pyramidal cells in the stratum lucidum . A broken puff pipette was positioned at ~20 μm from the thorny excrescence. Local delivery of MNI-Glutamate (10 mM, diluted in oxygenated ACSF) was achieved by low-pressure ejection of the solution (2 psi, 5 to 15 ms) using a PicoSpritzer III (Parker Instrumentation, NJ, USA). The laser wavelength was switched to 720 nm for two-photon photostimulation. To replicate glutamate release at multiple sites by mossy fibres, 10 individual points were positioned around a complex spine. Glutamate was liberated for 100 μs on individual points and the laser beam was rapidly redirected by acusto-optical deflectors AODs between points (6.5 μs), yielding a total time of <1.1 ms for a single stimulation event. Electrophysiological data were acquired in current-clamp mode. Glutamate uncaging was repeated 10 times at 20 Hz and at least 10 sweeps were obtained at 0.1 Hz for every cell. AP jitter was calculated using 8 ms window. Data analysis Synaptic events were analyzed using pClamp 10 software, individual events were detected using a template search and all were visually inspected to ensure appropriate kinetic properties. Events with multiple peaks and undetermined rising phase were excluded from analysis. Templates were created using the average of at least 10 events aligned by the rising of their slopes. Asynchronous release was estimated after 20 Hz stimulation train (10-stimuli train was repeated 10–30 times with 15–20 s interval). The number of all EPSCs was counted 200 ms after the last stimulus, within a 500-ms period. The sEPSCs was calculated before stimulation and used to correctly estimate aEPSCs using the following equation: aEPSCs=EPSCs−sEPSCs. Peak amplitude and kinetic properties of aEPSCs were measured only for cells with >60% of asynchronous events among all EPSCs (in average 75%). The peak amplitude of eEPSCs was measured for each individual response, and averaged and normalized to the first response. Recorded responses from the same cell were averaged, the decay tau was measured after the last stimulus, and the cumulative charge was measured either for ten individual responses (integral of 50 ms each) or in the whole response (integral of 1,000 ms total). In addition to aEPSCs frequency, cumulative charge was measured for the same time-window to estimate asynchronous release. PPR of EPSCs were determined using 20 Hz paired pulse stimulation protocol delivered with different time intervals varying from 10 s to 200 ms, which corresponds to basal stimulation frequencies from 0.1 to 5 Hz. Non-stationary variance–mean analysis was done using compound binomial equation: in which σ 2 is the variance, Q is the quantal size, N is the number of release sites and is the average EPSC amplitude. The coefficient of variation (CV) was measured as the s.d. of EPSCs ( σ ) divided by the mean ( μ ): CV= σ / μ and estimated for every cell. The variance–mean plots reached a plateau ( Supplementary Fig. 1A,B ) and the estimated maximum P at the end of the train was in the moderate range as defined in the study by Clements and Silver [68] (WT: P max =0.46±0.034, n =12; KO: 0.45±0.043, n =13). Therefore, the data could be reliably fitted with a compound binomial equation [68] . The convergence of parabolic fits was confirmed in each case using Igor Pro 6.2 software (Wavemetrics, Portland, OR, USA). To measure the RRP size, the sum of cumulative peak amplitude responses evoked by 3,000-stimuli 50 Hz train was calculated [40] . Deconvolution analysis was also done in IgorPro 6.2. We used a previously published deconvolution method; artificial miniature EPSCs (mEPSCs) were created using a rising phase of averaged mEPSCs recorded in TTX and a double exponential fit of decay to remove noise [46] . Separate artificial mEPSCs were used for each cell, amplitudes were not scaled. The cumulative synchronous release was calculated as an integral of release rate curve in a 10 ms time-window after each stimulus, and asynchronous release was calculated between 10 and 50 ms after stimuli. Current-clamp recordings were used to investigate the translation of presynaptic activity into postsynaptic firing. Cells were stimulated with four natural-like trains obtained from firing patterns of granule cells recorded in vivo (duration 8–24 s). Granule cell firing patterns were kindly provided by György Buzsáki (NYU) and were part of a previously published data [69] . A minimal inter-stimulus interval was 6 ms to ensure adequate action potential resolution. Each cell was stimulated with 1–3 different trains, repeated for 10 times with 20 s interval. The stimulation intensity was adjusted in voltage-clamp mode to evoke EPSCs with an average amplitude of 280±14 pA, this amplitude was sufficient to trigger action potentials in response to ~50% of stimuli. Responses were converted into binary files (0/1), corresponding to failure/success; double spikes in response to one stimulus were excluded from analysis (<1% of all spikes). Unstable responses with >20% change in the total number of spikes were not used for coherence and information. Binary files of responses and inter-stimulus intervals were used to quantify the amount of transferred information; this method was described in detail previously [48] . This analysis was performed with a code written in MATLAB software (MathWorks, Natick, MA, USA). Stimulus–response coherence C SR ( f ) was calculated from the cross-spectrum SR i ( f ) between the stimulus S and spike train R i ( i —repetition number, n –number of repetitions), the stimulus power spectrum SS( f ), and the power spectrum RR i ( f ) of spike train R i : Transferred information I ( f ) was calculated using following equation: The total information rate I was obtained by integrating I ( f ) between 0 and the maximal stimulus frequency 168 Hz. To compare the amount of information transfer between different cells total I was normalized to the average number of action potentials in response of the cell that gave us information per single postsynaptic AP. SR coherence was proposed by Roddey et al. [49] to estimate neuronal encoding performed by linear model. Given that neurons are non-linear systems, and could perform encoding more efficiently than described by any linear model, SR coherence corresponds to the best estimate of lower bound for information transfer. Upper bound of non-linear model performance could be calculated as the response–response (RR) coherence, C RR ( f ): Difference between the SR coherence and the square root of the RR coherence corresponds to the performance of the best linear model in comparison with the maximum theoretically achievable information coding. In addition, a more precise analysis of spike times was done by measuring time-to-peak for each evoked AP. Response delay was calculated as difference between stimulation time and time-to-peak within 6-ms window, except for the uncaging experiments, where 8-ms window was used. Jitter was calculated as s.d. of delay only for those responses, which had at least 4 APs evoked within 10 repetitions. Out of all responses analyzed for jitter, the majority (80%) included more than seven APs used to calculate s.d. Around 40% of all responses did not trigger sufficient number of APs for jitter calculation and were excluded from analysis. This statistic is based on the data set from in vivo stimulation experiments. In some cells, secondary APs were triggered, but occurred well outside 6 ms window and were not further analyzed. All plots were done using OriginPro7 software (OriginLab Corporation, Northampton, MA, USA). Data are expressed as mean±s.e.m. The statistical significance of differences was assessed with one or two-sample Student’s t -test. The level of significance was set at P <0.05. Electron microscopy Animals used for the electron microscopy were deeply anesthetized and transcardially perfused first with saline followed by 4% paraformaldehyde and 0.05% glutaraldehyde solution. Brains were removed from the skull and sectioned with a Vibratome at 50 μm. Free-floating sections were washed with Tris buffer (pH 7.4) for 5 min. Next, the sections were washed with Tris buffer for 5 min, then osmificated with 1% OsO 4 for 1 h, dehydrated and flat-embedded in Durcupan according to routine electron-microscopic procedure. After microscopic examination, the area of interest was cut, re-embedded and thin sectioned. Thin sections were stained with uranyl acetate and lead citrate. Tecnai electron microscope was used throughout the analysis. Vesicle density was calculated by manually counting vesicles in a randomly placed 500 × 500 nm square within presynaptic terminals. Vesicle density at various distances from the active zone was calculated in rectangles, where the base was parallel with the active zone and matched its length and the height was 50 nm. Vesicles within rectangles were counted manually. Docked vesicles were identified based on their tight juxtaposition with the presynaptic membrane and manually counted along the length of the active zone. All measurements were normalized, vesicle density was normalized to 1 μm 2 tissue area and the number of docked vesicles was normalized to a 100 nm long active zone. How to cite this article: Evstratova, A. et al. Vesicles derived via AP-3-dependent recycling contribute to asynchronous release and influence information transfer. Nat. Commun. 5:5530 doi: 10.1038/ncomms6530 (2014).